Complementary spin-Hall and inverse spin-galvanic effect torques in a ferromagnet/semiconductor bilayer Recently discovered relativistic spin torques induced by a lateral current at a ferromagnet/paramagnet interface are a candidate spintronic technology for a new generation of electrically controlled magnetic memory devices. The focus of our work is to experimentally disentangle the perceived two model physical mechanisms of the relativistic spin torques, one driven by the spin-Hall effect and the other one by the inverse spin-galvanic effect. Here, we show a vector analysis of the torques in a prepared epitaxial transition-metal ferromagnet/semiconductor-paramagnet single-crystal structure by means of the all-electrical ferromagnetic resonance technique. By choice of our structure in which the semiconductor paramagnet has a Dresselhaus crystal inversion asymmetry, the system is favourable for separating the torques due to the inverse spin-galvanic effect and spin-Hall effect mechanisms into the field-like and antidamping-like components, respectively. Since they contribute to distinct symmetry torque components, the two microscopic mechanisms do not compete but complement each other in our system. The two considered microscopic origins of the relativistic spin torques observed at a ferromagnet/paramagnet interface [1] , [2] have the following basic characteristics: in one picture, a spin current generated in the paramagnet via the relativistic spin-Hall effect [3] (SHE) is absorbed in the ferromagnet and induces the spin transfer torque [4] (STT). In the other picture, a non-equilibrium spin-density is generated via the relativistic inverse spin-galvanic effect [5] (ISGE) and induces the spin–orbit torque [6] , [7] , [8] (SOT) in the ferromagnet. From the early observations in paramagnetic semiconductors, SHE and ISGE are known as companion phenomena that can both allow for electrically aligning spins in the same structure [9] , [10] , [11] . It is therefore both challenging and desirable for our basic physical understanding of the spin torques at the ferromagnet/paramagnet interface to experimentally disentangle the SHE and ISGE contributions. The splitting of the two microscopic mechanisms between the field-like and the antidamping-like torque components has not been previously achieved for several conceptual reasons. The original theoretical proposals [12] , [13] , [14] and experimental observations [10] , [11] , [15] , [16] of the ISGE were made in paramagnets with no ferromagnetic component in the structure. The corresponding non-equilibrium spin density, generated in the ISGE by inversion-asymmetry terms in the relativistic Hamiltonian, has naturally no dependence on magnetization. Hence, in the context of magnetic semiconductors [6] , [8] , [17] , [18] or ferromagnet/paramagnet structures [1] , [7] , [19] , [20] , [21] , the ISGE may be expected to yield only the field-like component of the torque ~ M × ζ , where the vector ζ is independent of the magnetization vector M (see Fig. 1a ). However, when carriers experience both the spin–orbit coupling and magnetic exchange coupling, the inversion asymmetry can generate a non-equilibrium spin density component of extrinsic, scattering-related [22] , [23] or intrinsic Berry-curvature [24] , [25] , [26] origin, which is magnetization dependent and yields an antidamping-like torque ~ M × ( M × ζ ). Experiments in (Ga,Mn)As confirmed the presence of the ISGE-based mechanism [8] , [17] , [18] and demonstrated that the field-like and the Berry-curvature antidamping-like SOT components can have comparable magnitudes [25] . 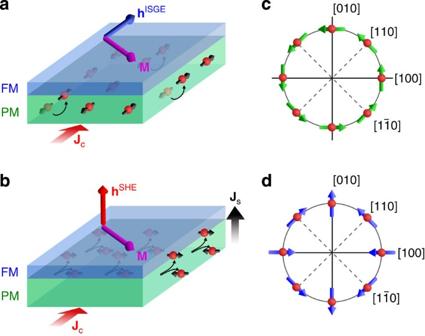Figure 1: Microscopic origins of the SHE and ISGE torques (a) In the paramagnetic GaAs layer (PM), as charge carriers are accelerated by an applied electric field in the inversion-asymmetric crystal potential, scattering events lead to a non-equilibrium spin polarization. The spin polarization depends on the direction of the current with respect to crystal direction. Through exchange coupling at the interface, the magnetization,M, in the ferromagnetic layer (FM) experiences an effective field,hISGE, parallel to the spin polarization. (b) In the GaAs layer, when a longitudinal charge current,Jc, is applied, a transverse spin current,Js, is induced by the SHE, which flows into the Fe layer. The spin current exerts a torque that depends on the magnetization angle. For an in-plane magnetization this is described by an out-of-plane effective field,hSHE. (c) In transition-metal bilayers, only a Rashba-symmetry spin polarization may be generated by the structural inversion asymmetry. (d) In GaAs, the spin polarization of the ISGE has the Dresselhaus symmetry for carrier momentum in different crystal directions. Figure 1: Microscopic origins of the SHE and ISGE torques ( a ) In the paramagnetic GaAs layer (PM), as charge carriers are accelerated by an applied electric field in the inversion-asymmetric crystal potential, scattering events lead to a non-equilibrium spin polarization. The spin polarization depends on the direction of the current with respect to crystal direction. Through exchange coupling at the interface, the magnetization, M , in the ferromagnetic layer (FM) experiences an effective field, h ISGE , parallel to the spin polarization. ( b ) In the GaAs layer, when a longitudinal charge current, J c , is applied, a transverse spin current, J s , is induced by the SHE, which flows into the Fe layer. The spin current exerts a torque that depends on the magnetization angle. For an in-plane magnetization this is described by an out-of-plane effective field, h SHE . ( c ) In transition-metal bilayers, only a Rashba-symmetry spin polarization may be generated by the structural inversion asymmetry. ( d ) In GaAs, the spin polarization of the ISGE has the Dresselhaus symmetry for carrier momentum in different crystal directions. Full size image The STT is dominated by the antidamping-like component [4] in weakly spin–orbit-coupled ferromagnets with τ ex ≪ τ s , where τ ex is the precession time of the carrier spins in the exchange field of the ferromagnet and τ s is the spin lifetime in the ferromagnet. This, in principle, applies also to the case when the spin current is injected to the ferromagnet from a paramagnet via the SHE (see Fig. 1b ). However, at finite τ s , the STT also acquires a field-like component [4] . Experiments in W/Hf/CoFeB structures confirmed the presence of the SHE-based mechanism in the observed torques and showed that the SHE–STT can have both antidamping-like and field-like components of comparable magnitudes [27] . In the commonly studied polycrystalline transition-metal ferromagnet/heavy-metal paramagnet samples, the dependence of the torques on the angle of the driving in-plane current also does not provide the direct means to disentangle the two microscopic origins. The lowest-order inversion-asymmetry spin–orbit terms in the Hamiltonian have the Rashba form (see Fig. 1c ) for which the vector ζ is in the plane parallel to the interface and perpendicular to the current, independent of the current direction. The same applies to the spin polarization of the SHE spin current propagating from the paramagnet to the ferromagnet. The M and ζ functional form of the field-like and antidamping-like SHE–STTs is the same as of the corresponding SOT components. In the observed lowest-order torque terms in Pt/Co and Ta/CoFeB structures [28] , the ISGE-based and the SHE-based mechanism remained, therefore, indistinguishable. The simultaneous observation of higher-order torque terms in these samples pointed to SOTs due to structural inversion-asymmetry terms beyond the basic Rashba model. From the Ta thickness dependence measurements in the Ta/CoFeB structure, it was concluded that in these samples both the ISGE-based and the SHE-based mechanisms contributed to both the field-like and the antidamping-like torques [29] . The SHE and ISGE were originally discovered in III–V semiconductors [9] , [10] , [11] , [15] , [16] but for maximizing the relativistic spin torques in common transition-metal ferromagnets, it turned out to be more suitable to interface them with the highly conductive heavy-metal paramagnets such as Pt, Ta or W [1] , [2] , [27] , [28] , [29] . To clearly separate the two microscopic origins of the torques, returning to III–V semiconductor paramagnets is instrumental as the leading inversion-asymmetric term is played by the broken inversion symmetry in the crystal structure. Independent of the interface, holes in the strained zinc-blende lattice of a III–V semiconductor experience a linear-in-wavevector Dresselhaus spin–orbit coupling. The ISGE of the corresponding symmetry (see Fig. 1d ) generated in the semiconductor should induce a SOT in an adjacent ferromagnetic film with ζ perpendicular to the current for current along [110] or crystal axes of the semiconductor, while ζ should be parallel to the current for the [100] or [010] current directions. In the following, we measure the relativistic spin torques in a single crystal Fe (2 nm)/(Ga,Mn)As (20 nm) bilayer using an electrically induced and detected ferromagnetic resonance (FMR) technique [18] , [30] (for growth details see Methods). We dope the GaAs host with ~3% of substitutional Mn Ga acceptors to increase the semiconductor conductivity, while not providing a sizeable exchange splitting within the semiconductor at room temperature. From magnetization angle dependence measurements of the FMR voltages, we find the field-like and antidamping torques have similar magnitudes. By measuring devices where the current is along different crystal directions of the semiconductor, we show that the ISGE with a characteristic Dresselhaus symmetry induces only the field-like torque in the adjacent Fe, whereas the SHE spin current, generated inside the paramagnetic p-doped GaAs layer, is absorbed in the weakly spin–orbit-coupled Fe in the form of the antidamping-like STT. Therefore in this bilayer, we show that the ISGE and SHE mechanisms are separated into distinct symmetry components of the current-induced torque. Electrically-induced FMR measurements Current-induced torques were measured in patterned bars of width 10μm and length 200μm using an all-electrical FMR technique (see Fig. 2a ). In this method, a microwave current flowing in the device induces FMR when the externally applied magnetic field matches the resonant condition. The resonance of the Fe magnetization is detected in the d.c. voltage induced across the bar, V d.c. . This is due to the homodyne mixing of the microwave current with the oscillating component of magnetoresistance caused by the magnetization precession. In these measurements, we increase the microwave current coupled into the sample, with a typical resistance of 8 kΩ, using an impedance matching network [30] (see Methods and Supplementary Note 1 ). 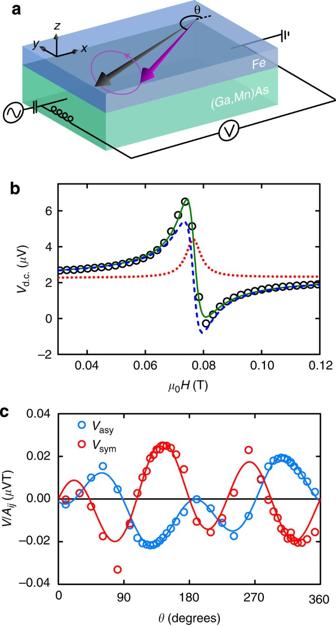Figure 2: Electrical excitation and detection of FMR (a) Schematic of the measurement showing magnetization precession. A microwave current passes through the capacitor of the bias-T and into the Fe/GaAs bilayer sample where the current-induced torques causes the magnetization of the Fe (purple arrow) to precess around the external field (black arrow). The precession is detected in the d.c. voltage measured across the device by a magnetoresistance mixing effect. (b) A typical FMR curve is detected inVd.c.(data points) as a function of external field, induced by a 16.245GHz microwave current.Vd.c.is fitted (solid green line) by a combination of symmetric (red dotted line) and antisymmetric (blue dashed line) Lorentzians. (c) The in-plane magnetization angle dependence of the fitted Lorentzian amplitudes for a device with current in the [010] crystal direction. Figure 2: Electrical excitation and detection of FMR ( a ) Schematic of the measurement showing magnetization precession. A microwave current passes through the capacitor of the bias-T and into the Fe/GaAs bilayer sample where the current-induced torques causes the magnetization of the Fe (purple arrow) to precess around the external field (black arrow). The precession is detected in the d.c. voltage measured across the device by a magnetoresistance mixing effect. ( b ) A typical FMR curve is detected in V d.c. (data points) as a function of external field, induced by a 16.245GHz microwave current. V d.c. is fitted (solid green line) by a combination of symmetric (red dotted line) and antisymmetric (blue dashed line) Lorentzians. ( c ) The in-plane magnetization angle dependence of the fitted Lorentzian amplitudes for a device with current in the [010] crystal direction. Full size image For a series of external magnetic field directions in the plane of the sample, FMR sweeps were recorded using a microwave frequency of close to 16 GHz. From the magnetization angle dependence of the resonance field, we obtained the magnetization amplitude value of μ 0 M s =1.85±0.03 T, which is close to the literature value of 1.7 T for Fe [31] , and we found an in-plane uniaxial anisotropy of μ 0 H U =0.101±0.001 T, which is typical for thin films of Fe grown on GaAs [32] . By solving the Landau–Lifshitz–Gilbert equation for a small current-induced excitation field, ( h x , h y , h z ) e jωt , V d.c. is found to be comprised of symmetric and antisymmetric Lorentzian functions with coefficients V sym and V asy , respectively. Here h x is the excitation field component parallel to the current and h y is the component perpendicular to the current. h z is the component perpendicular to the plane of the bilayer. The coefficients depend on the angle, θ , of the magnetization vector relative to the current and are given by Here, V mix is the sensitivity of the mixing detection and is given by , where I 0 ( e jωt , 0, 0) is the microwave current in the device and Δ R is the coefficient of the anisotropic magnetoresistance of the sample. A yy and A yz are the diagonal and off-diagonal components of the a.c. magnetic susceptibility, which depend on the magnetic anisotropies and Gilbert damping of the sample. In our devices, Δ R is typically 17 Ω which, assuming Fe carries the majority of the current in the bilayer, is consistent in sign and magnitude with literature values of 0.2% anisotropic magnetoresistance in Fe [33] . We estimate the proportion of total bilayer current in the Fe layer to be 79% by resistance measurements of Hall bars before and after removing the Fe and capping Al (see Supplementary Note 2 ). FMR measurements were made using devices patterned in four crystal directions. The microwave power for all devices, incident on the impedance matching network, was 24 dBm. For each angle, the resonances were fitted by symmetric and antisymmetric Lorentzian functions. A typical curve is shown in Fig. 2b . The in-plane uniaxial magnetic anisotropy of Fe implies that, in general, the magnetization does not lie along the external field. The actual magnetization angles and uniaxial anisotropy are self-consistently calculated from the dependence of the resonant field on the external magnetic field angle [34] . This also allows the susceptibilities, A yz and A yy , to be calculated. The magnetization angle dependence of V sym / A yz and V asy / A yy is plotted in Fig. 2c for a bar patterned in the [010] crystal direction. The full expression for the angle dependence of the fitted data is given in Supplementary Note 3 . Validity of FMR analysis Our analysis of the current-induced torques using equation (1) is not necessarily valid if the torques do not act in phase with the microwave current. In comparison with electrically detected FMR measurements where the microwave current is capacitively or inductively coupled into the sample [35] , we do not expect a phase-shift between the microwave current and induced fields as the current is conducted ohmically. Nevertheless, we might worry that some part of our microwave resonator circuit leads to a phase shift. To test this, we repeated our measurements with a [100] device over a frequency range (11.8–14.4 GHz) using a microstrip resonator with a fundamental frequency close to 13 GHz ( Fig. 3a ). If there were some frequency-dependent phase shift, we would expect the lineshape to oscillate between an antisymmetric and symmetric Lorentzian over this frequency range. However, the ratio of V sym to V asy remains constant in this frequency range to within experimental error ( Fig. 3b ), confirming that our analysis is correct. 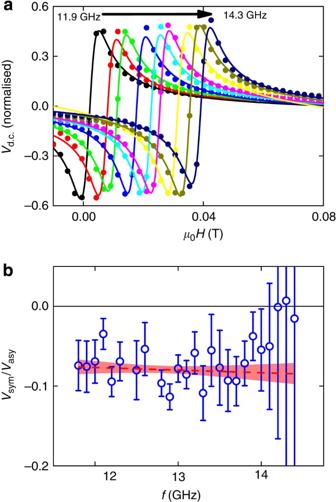Figure 3: Frequency independence of the FMR lineshape (a) Normalized, fitted, resonant peaks for a series of microwave frequencies detected inVd.c.. The lineshape is dominated by an antisymmetric Lorentzian for every frequency. (b) The ratio ofVsymtoVasy(blue circles) is constant to within the standard error (red shaded region) of a linear fit (red dashed line) for the measured frequency range. The error in the ratio is bigger away from the impedance-matched frequency (13 GHz) of the microstrip resonator used, as the detected peak inVd.c.is smaller. Figure 3: Frequency independence of the FMR lineshape ( a ) Normalized, fitted, resonant peaks for a series of microwave frequencies detected in V d.c. . The lineshape is dominated by an antisymmetric Lorentzian for every frequency. ( b ) The ratio of V sym to V asy (blue circles) is constant to within the standard error (red shaded region) of a linear fit (red dashed line) for the measured frequency range. The error in the ratio is bigger away from the impedance-matched frequency (13 GHz) of the microstrip resonator used, as the detected peak in V d.c. is smaller. Full size image Analysis of the current-induced torques As shown in Fig. 4a , the in-plane current-induced field depends strongly on the crystal direction of the current and can be well fitted by the Dresselhaus symmetry ISGE field, h ISGE ~(cos 2 φ [100] , −sin 2 φ [100] , 0), where φ [100] is the angle between the current and the [100] crystal direction. This is the expected symmetry of the current-induced non-equilibrium spin polarization of carriers in the semiconductor due to the inversion-asymmetric crystal structure of the strained zinc-blende lattice of (Ga,Mn)As. The interface exchange coupling of these polarized carriers with the adjacent Fe moments induces the field-like SOT in Fe with the Dresselhaus symmetry. We note that other torque terms with the symmetry common to the Rashba ISGE, the field-like component of the SHE–STT or the torque due to an Oersted field have only a minor contribution to the total measured field-like torque. 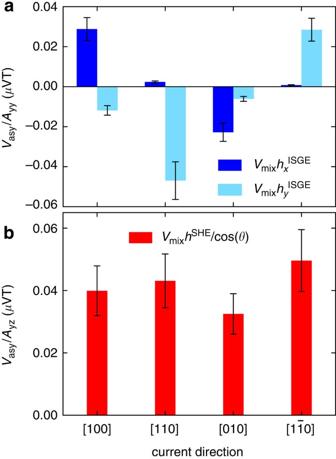Figure 4: Dependence of the effective fields on the crystal direction of the current (a) The fitted in-plane field coefficients for a set of devices in different crystal directions. (b) The fitted out-of-plane field coefficient (representing the antidamping torque) for the same devices. Error bars shown are calculated by estimating the standard deviation inVmixdue to the variance in the calibration of the microwave current. Figure 4: Dependence of the effective fields on the crystal direction of the current ( a ) The fitted in-plane field coefficients for a set of devices in different crystal directions. ( b ) The fitted out-of-plane field coefficient (representing the antidamping torque) for the same devices. Error bars shown are calculated by estimating the standard deviation in V mix due to the variance in the calibration of the microwave current. Full size image To highlight that carriers in the semiconductor layer are responsible for the Dresselhaus symmetry ISGE field, we compare Fig. 4a with previous measurements in which the in-plane current-induced fields were measured in a bare (Ga,Mn)As epilayer [25] without the Fe film. To observe the corresponding SOT in this sample, a larger concentration of magnetic Mn moments was used, and the measurements were performed at low temperatures where the Mn moments are ferromagnetic in equilibrium. Instead of the interfacial exchange coupling to Fe, the current-induced non-equilibrium spin polarization of carriers in the semiconductor due to the Dresselhaus symmetry ISGE is exchange-coupled directly to the ferromagnetic moments on which it exerts the field-like SOT. In both the Fe/(Ga,Mn)As and the (Ga,Mn)As samples the same crystal-symmetry field-like SOT is observed, which confirms their common Dresselhaus ISGE origin. In contrast to the in-plane field, the out-of-plane current-induced field is independent of the crystal direction of the current but depends on the magnetization angle. It is dominated by a term h SHE ~ M × y ( y is the direction transverse to the current), which generates the antidamping-like torque. As shown in Fig. 4b , the amplitudes of the field-like and antidamping-like torques are comparable in our Fe/(Ga,Mn)As structure. The underlying microscopic mechanism of the antidamping component can only be of the SHE–STT origin. The experimental error shown in Fig. 4b is greater than any crystal-dependent variation in the spin-Hall angle. In previous measurements in the bare (Ga,Mn)As epilayer [25] , the antidamping-like SOT was dominated by the counterpart microscopic mechanism to the Dresselhaus ISGE. This Dresselhaus-symmetry antidamping-like SOT is clearly missing in our measured data. It is suppressed in our Fe/(Ga,Mn)As structure by design, because carriers in the semiconductor are not sufficiently magnetized at equilibrium due to the low Mn moment density and high temperature of the experiment. In principle, one might also consider that the spin accumulation induced by the Dresselhaus ISGE could cause a diffusive spin current to flow into the ferromagnet and exert an antidamping-like STT. This would have the Dresselhaus symmetry that is, however, not seen in our antidamping-like torque data. A Rashba-symmetry antidamping-like SOT due to the carriers in the Fe experiencing the inversion asymmetry of the interface could in principle also explain the symmetry of our data; however, we do note the lack of a corresponding strong Rashba-symmetry field-like SOT. This antidamping SOT would have the same symmetry as the antidamping SHE–STT. This possibility is, however, ruled out by our control experiment in which we perform electrically detected FMR in a similar molecular beam epitaxy-grown Fe (1 nm)/insulating GaAs structure at room temperature. In this case, we do not observe the antidamping torque in the rectification effect, despite the sample possessing a similar magnetoresistance ratio (~0.2%) to our Fe/(Ga,Mn)As. This is consistent with the carriers being removed from the semiconductor, which eliminates the SHE source of the spin current. We note that also consistently with the absence of carriers in the semiconductor in the Fe/insulating GaAs structure, we do not observe the Dresselhaus-symmetry field-like SOT in this control sample. Determining the magnitudes of the ISGE and SHE To calibrate the microwave current in the sample we used a bolometric technique (see Supplementary Fig. 1 and Supplementary Note 4 ). Using this calibration, we estimate amplitudes of | μ 0 h ISGE / J GaAs |=16±10 μT per 10 6 A cm −2 and | μ 0 h SHE / J GaAs |=20±9 μT per 10 6 A cm −2 . The error is found from the statistical variation of all of the devices measured. To verify the bolometric calibration, we also perform an additional check with a single device by measuring the change in Q -factor of the microstrip resonator loaded with and without a sample (see Supplementary Figs 2 and 3 and Supplementary Note 5 ). This calibration yields values of | μ 0 h ISGE / J GaAs |=37 μT per 10 6 A cm −2 and | μ 0 h SHE / J GaAs |=47 μT per 10 6 A cm −2 , close to the values of the bolometric technique. From the measured h SHE in our Fe/(Ga,Mn)As structure we can infer the room-temperature spin-Hall angle, θ SH , in the paramagnetic (Ga,Mn)As using the expression based on the antidamping-like STT [2] , Here it is assumed that the thickness of the semiconductor is much larger than its spin diffusion length (5.6 nm in p-GaAs [36] ) and d Fe is the thickness of the Fe layer. Equation (2) yields values of θ SH =1.7±0.9% (bolometric calibration) and 4% ( Q -factor calibration), similar to spin-Hall angles previously reported for carriers with a p-orbital character in GaAs [36] , [37] . This agreement with previously measured spin-Hall angles is further evidence that the antidamping-like torque does not have a significant Rashba-symmetry SOT contribution. To check these spin-Hall values, we compare our torque efficiencies in terms of field per total current density with those of transition metal/ferromagnet bilayers. For instance, Garello et al. [28] measured an antidamping-like torque of | μ 0 h / J |=690 μT per 10 6 A cm −2 in layers with 0.6 nm Co and 3 nm Pt and an equivalent spin-Hall angle of 16%. Although our spin-Hall angle is only 4–8 times smaller, the field per total current density is 85–170 times smaller because the total magnetic moment of our Fe layer is ~4 times higher than of the Co and ~80% of the total current is shunted through the Fe. To conclude, we have experimentally disentangled the two archetype microscopic mechanisms that can drive relativistic current-induced torques in ferromagnet/paramagnet structures. In our epitaxial Fe/(Ga,Mn)As bilayer we simultaneously observed ISGE-based and SHE-based torques of comparable amplitudes. Designed magnetization-angle and current-angle symmetries of our single-crystal structure allowed us to split the two microscopic origins between the field-like and the antidamping-like torque components. Experimentally establishing the microscopic physics of the relativistic spin torques should stimulate both the fundamental and applied research of these intriguing and practical spintronic phenomena. Thin-film growth To obtain measurable torques in a metal-ferromagnet/semiconductor-paramagnet structure requires at least partially matched conductances of the semiconductor and metal layers, which we achieved by doping a GaAs host with ~3% of substitutional Mn Ga acceptors. Mn allows us to achieve this exceptionally high charge-doping. The semiconductor (Ga,Mn)As layer of thickness 20 nm was deposited on a GaAs(001) substrate by molecular beam epitaxy at a temperature of 260 °C. The substrate temperature was then reduced to 0 °C, before depositing a 2-nm Fe layer, plus a 2-nm Al capping layer without breaking vacuum. In situ reflection high-energy electron diffraction and ex situ X-ray reflectivity and diffraction measurements confirmed that the layers are single crystalline with sub-nm interface roughness. Impedance matching To improve the sensitivity of the FMR measurement, the sample is embedded in a microstrip resonator circuit [30] , which acts to impedance match the ~8-kΩ sample to the external 50-Ω transmission line at the fundamental frequency (in this case ~8 GHz) or harmonic frequencies of the resonator (see Supplementary Note 1 ). To allow measurement of V d.c. , the resonator contains an on-board bias-T. In this experiment, FMR measurements are made at the the 2nd harmonic frequency of the resonator (~16 GHz). How to cite this article: Skinner, T. D. et al. Complementary spin-Hall and inverse spin-galvanic effect torques in a ferromagnet/semiconductor bilayer. Nat. Commun. 6:6730 doi: 10.1038/ncomms7730 (2015).